Lagrangian scale of particle dispersion in turbulence Transport of mass, heat and momentum in turbulent flows by far exceeds that in stable laminar fluid motions. As turbulence is a state of a flow dominated by a hierarchy of scales, it is not clear which of these scales mostly affects particle dispersion. Also, it is not uncommon that turbulence coexists with coherent vortices. Here we report on Lagrangian statistics in laboratory two-dimensional turbulence. Our results provide direct experimental evidence that fluid particle dispersion is determined by a single measurable Lagrangian scale related to the forcing scale. These experiments offer a new way of predicting dispersion in turbulent flows in which one of the low energy scales possesses temporal coherency. The results are applicable to oceanographic and atmospheric data, such as those obtained from trajectories of free-drifting instruments in the ocean. In problems such as spreading of plankton in the ocean, transport of pollutants in the atmosphere, mixing of fluids or rain initiation in clouds, the understanding of statistical properties of Lagrangian trajectories in turbulence is crucial.The relationship between descriptions of turbulence from the point of view of a still observer (Eulerian description) and that of a particle moving with the flow (Lagrangian description) remains unresolved in the theory of turbulence [1] . Recent advances in numerical modelling and experimental particle tracking in turbulence [2] greatly improved our understanding of Lagrangian trajectories [3] , [4] , [5] . The most basic property of Lagrangian trajectories is a single-particle dispersion, or mean-squared displacement, of a particle moving along the trajectory from its initial position . Einstein predicted ballistic and diffusive transport at short and large times, respectively, for Brownian particles [6] . In turbulence, single-particle dispersion is governed by the stochastic equation, and, as has been shown by Taylor [7] , it is similar to the Einstein's theory of Brownian motion: Here u is the particle velocity, is the Lagrangian integral time, which can be obtained from the Lagrangian velocity autocorrelation function, where is the velocity variance. To estimate the diffusion coefficient D exp =‹ u 2 › T L at large times, one needs to compute, or to measure, the Lagrangian velocity correlation function. The problem however is that ρ ( t ) and T L cannot be theoretically predicted and their relationship with their Eulerian counterparts is still debated. For example, some authors expect that the Lagrangian correlation time should be larger than the Eulerian time, T L / T E >1 (ref. 8 ), as in fact has been found in some atmospheric measurements [9] , while the theoretical analysis by Middleton [10] gave a different result, T L / T E <1. In addition to the Lagrangian integral time T L , it is common to use the Lagrangian integral scale L L , and it is often assumed (for example, Lumpkin et al . [11] ) that as the Lagrangian particle moves at a characteristic speed , the Lagrangian integral time and space are related as We will show that L L can be used to determine the diffusivity: This diffusivity, equation (5), is often estimated using a typical magnitude of the horizontal eddy velocity, and the mixing length L . It is usually expected that larger and more energetic eddies will be dominant contributors to the eddy diffusivity [12] . We report on the measurements of Lagrangian characteristics in two-dimensional (2D) turbulence. Experiments have been conducted in both underdeveloped (chaotic) and in fully developed turbulent flows to measure dispersion in a broad range of the flow kinetic energies, driven at different forcing scales. To investigate particle dispersion in both ballistic regime, equation (1), and in diffusive regime, equation (2), floating tracer particles in the flow are tracked with high-resolution for sufficiently long time. In the reported experiments we show that it is the most coherent scale, rather than the energy-containing scale, which determines L L . Characteristics of turbulent flows Experiments are performed by using two very different methods of turbulence generation. In the first, turbulence is excited electromagnetically [13] , [14] (electromagnetically driven turbulence (EMT)). In the second set of experiments, 2D turbulence is driven by Faraday waves on the surface of a vertically vibrated fluid container (Faraday wave driven turbulence (FWT)), a method which just recently has been discovered in von Kameke et al . [15] and further investigated in Francois et al . [16] The tracer particles on the water surface are accelerated in the wave field and move chaotically in the horizontal plane. Though the vertical motion is also present on the rippled surface, statistics of the horizontal velocity fluctuations are fully consistent with those in 2D turbulence. Both experiments have distinct advantages. FWT can be produced in a broad range of forcing levels (vertical accelerations) and forcing scales (by changing the vibration frequency), while the electromagnetically driven scheme produces both regular and turbulent flows ( Fig. 1a–d ). 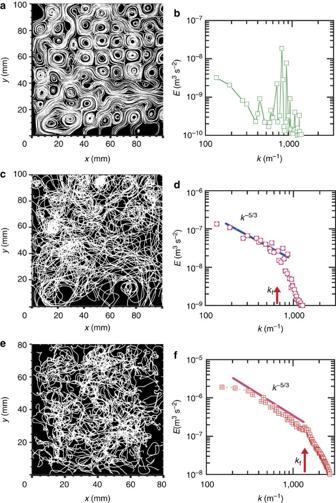Figure 1: Particle trajectories and kinetic energy spectra in different flows. (a) If the flow is weakly forced electromagnetically (the current density of 0.2 × 103A m−2here), the forcing scale vortices interact rather weakly, yet particles travel randomly in the box. (b) The spectral energy is localized in a narrow wave number range at aboutkf. (c) At higher forcing levels (the current density here is 1 × 103A m−2) particle trajectories are no longer dominated by the forcing scale vortices. (d) The energy spectrum spreads towards larger scales forming a continuous Kolmogorov–Kraichnan spectrum via the inverse energy cascade17Ek=Cε2/3k−5/3atk<kf. (e) Particles moving horizontally on the surface of parametrically driven Faraday waves show many characteristics of 2D turbulence, such as kinetic energy spectra, energy flux and particle dispersion. (f) A spectrum is shown for the value of the vertical acceleration ofa=1.6g. Figure 1: Particle trajectories and kinetic energy spectra in different flows. ( a ) If the flow is weakly forced electromagnetically (the current density of 0.2 × 10 3 A m −2 here), the forcing scale vortices interact rather weakly, yet particles travel randomly in the box. ( b ) The spectral energy is localized in a narrow wave number range at about k f . ( c ) At higher forcing levels (the current density here is 1 × 10 3 A m −2 ) particle trajectories are no longer dominated by the forcing scale vortices. ( d ) The energy spectrum spreads towards larger scales forming a continuous Kolmogorov–Kraichnan spectrum via the inverse energy cascade [17] E k = C ε 2/3 k −5/3 at k<k f . ( e ) Particles moving horizontally on the surface of parametrically driven Faraday waves show many characteristics of 2D turbulence, such as kinetic energy spectra, energy flux and particle dispersion. ( f ) A spectrum is shown for the value of the vertical acceleration of a =1.6 g . Full size image Regardless of the method of turbulence generation, spectra show the inverse energy cascade range [17] E k = Cε 2/3 k −5/3 at wave numbers k<k f , where k f is the forcing wave number, and ε is the energy dissipation rate. At larger wave numbers, k > k f , in the direct enstrophy cascade, the spectrum should scale as . In fact, spectra in Fig. 1d are steeper, , due to higher damping at large wave numbers [16] , [18] ; however, when turbulence is forced at lower wave numbers, for example, at f 0 =30 Hz in FWT, a theoretically predicted k −3 spectrum is observed in the enstrophy cascade range. The kink in the spectrum marks the forcing scale L f =2 π / k f . Temporal Lagrangian velocity autocorrelation The mean-squared dispersion of a tracer particle from the initial point on its trajectory is computed by averaging over two to three thousands of trajectories obtained using particle tracking velocimetry, such as those in Fig. 1 . The dispersion is shown as a function of time in Fig. 2a for the Faraday wave driven turbulence (the forcing scale of L f ≈4.4 mm). At shorter times, less than the Lagrangian integral time, t < T L , a clear ballistic regime is observed, , in agreement with Equation (1), while at larger times, we find a diffusive regime ‹ δr 2 ›≈2 D exp t , similar to recent observations [15] , [19] . Here we confirm these two regimes for a broad range of forcing levels, including the ‘underdeveloped’ turbulence, like for example, the one shown in Fig. 1a . The diffusion coefficient D exp , given by half the slope of the dispersion curve, increases when the forcing level is increased ( Fig. 2b ). This is true in both the Faraday wave driven and in EMT. However, when the mean-squared dispersions are plotted versus normalized time, t / T L ( Fig. 2c ), all dispersion curves of the Faraday wave driven turbulence for a given forcing scale collapse onto one. This suggests that the quantity is independent of the turbulence kinetic energy, where . It has a dimension of L 2 and this result points to the existence of a universal spatial scale of particle dispersion related to the forcing scale. 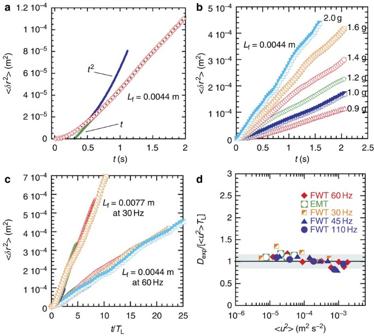Figure 2: Particle dispersion in 2D turbulence. (a) Statistically averaged mean-squared displacement of particles away from the initial position shows a ballistic regimeat short time shifts, and diffusive regimeat large times, in agreement with Einstein's and Taylor's results (equations 1, 2). Such particle dispersion is observed in all experiments presented in the paper. (b) Large time mean-squared displacements in the FWT. Turbulence is driven by vertically shaking the fluid cell at the frequency of 60 Hz at different vertical accelerations, from 0.9 to 2 g. The forcing scale isLf=4.4 mm. Increasing slopes of the curves are indicative of increasing diffusivity with forcing. (c) Mean-squared displacement curves at different forcing levels are plotted versus time shift normalized by the Lagrangian integral time,t/TL. These are shown for two sets of experiments,Lf=4.4 mm andLf=7.7 mm. This reveals constancy of, indicating that particle dispersion in turbulence universally depends on one characteristic scale,. (d) Particle diffusivities obtained from the slopes ofcurves are normalized by the product of the velocity variance and the corresponding integral time scale. Data points obtained in all experiments are plotted versus corresponding flow energies. All points converge to a value of. The shaded box shows the s.d. of the measurements. Figure 2: Particle dispersion in 2D turbulence. ( a ) Statistically averaged mean-squared displacement of particles away from the initial position shows a ballistic regime at short time shifts, and diffusive regime at large times, in agreement with Einstein's and Taylor's results (equations 1, 2). Such particle dispersion is observed in all experiments presented in the paper. ( b ) Large time mean-squared displacements in the FWT. Turbulence is driven by vertically shaking the fluid cell at the frequency of 60 Hz at different vertical accelerations, from 0.9 to 2 g. The forcing scale is L f =4.4 mm. Increasing slopes of the curves are indicative of increasing diffusivity with forcing. ( c ) Mean-squared displacement curves at different forcing levels are plotted versus time shift normalized by the Lagrangian integral time, t / T L . These are shown for two sets of experiments, L f =4.4 mm and L f =7.7 mm. This reveals constancy of , indicating that particle dispersion in turbulence universally depends on one characteristic scale, . ( d ) Particle diffusivities obtained from the slopes of curves are normalized by the product of the velocity variance and the corresponding integral time scale. Data points obtained in all experiments are plotted versus corresponding flow energies. All points converge to a value of . The shaded box shows the s.d. of the measurements. Full size image We performed over 30 experiments at different forcing levels (over three orders of magnitude in kinetic energy) and different forcing scales L f =(3.6–9) mm. In all conditions the ratio of the experimental diffusion coefficient D exp over the product is close to 1, Fig. 2d , confirming equation (2). Spatial Lagrangian velocity autocorrelation To detect this distinct Lagrangian scale we compute the spatial Lagrangian velocity autocorrelation function, which can be constructed similarly to the temporal autocorrelation function, equation (3): The Lagrangian integral scale is given by . Moving along a trajectory, we simultaneously record a particle's velocity and its displacement δr ( t ) from the initial position r 0 . By excluding time, we first interpolate measured velocity increments onto a regular array , and then compute the spatial autocorrelation function ρ ( L ). The Lagrangian velocity autocorrelation time T L decreases with the increase in the energy input, Fig. 3a , however, the Lagrangian integral scale L L is very weakly dependent on the forcing. For a given forcing scale in fully developed turbulence, spatial Lagrangian velocity autocorrelation functions ρ ( L ) approximately collapse onto each other, as illustrated in Fig. 3b . In all experiments, particle dispersion in 2D turbulence is determined by the Lagrangian autocorrelation scale and the r.m.s. velocity, , Fig. 3c . Turbulence accumulates energy in the inertial range and determines , while the Lagrangian scale L L determines the mean free path between the particle's memory loss events. 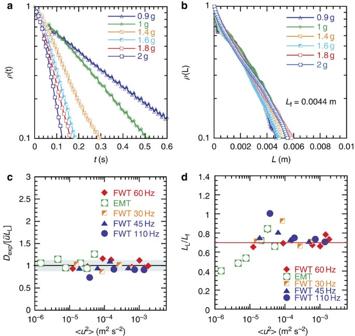Figure 3: Lagrangian characteristics of turbulent flows. (a) Temporal Lagrangian autocorrelation function, computed for a range of forcing levels in the FWT. This function is decaying approximately exponentially,, whereTLis Lagrangian integral time. (b) Spatial Lagrangian autocorrelation functioncomputed for the same conditions. As the turbulence energy is increased, Lagrangian integral length remains roughly constant in the broad range of forcing levels. (c) Fluid particle diffusivities normalized by the product of the square root of the velocity variance and the corresponding Lagrangian integral scale. Data points obtained in all experiments are plotted versus corresponding flow energies. All points converge to a value of. The shaded box shows the s.d. of the measurements. (d) The ratio of the Lagrangian integral scale and the corresponding forcing scaleLL/Lf. Figure 3: Lagrangian characteristics of turbulent flows. ( a ) Temporal Lagrangian autocorrelation function , computed for a range of forcing levels in the FWT. This function is decaying approximately exponentially, , where T L is Lagrangian integral time. ( b ) Spatial Lagrangian autocorrelation function computed for the same conditions. As the turbulence energy is increased, Lagrangian integral length remains roughly constant in the broad range of forcing levels. ( c ) Fluid particle diffusivities normalized by the product of the square root of the velocity variance and the corresponding Lagrangian integral scale. Data points obtained in all experiments are plotted versus corresponding flow energies. All points converge to a value of . The shaded box shows the s.d. of the measurements. ( d ) The ratio of the Lagrangian integral scale and the corresponding forcing scale L L / L f . Full size image The main error in the determination of either the ratio in Fig. 2d , or the ratio in Fig. 3c , comes from the integration of the autocorrelation functions ρ ( t ) or ρ ( L ) over the inevitably limited temporal or spatial domain. The error bar for L L and T L is ~10%. The error analysis of T L has been discussed in detail in Lumpkin et al . [11] In experiments at different forcing scales, the Lagrangian integral scale L L roughly follows the scale of forcing, Fig. 3d . The analysis of all experiments shows that the ratio of the Lagrangian integral scale and the scale of forcing, L L / L f , varies in the range from 0.4 to 1 in a broad range of conditions. This scale is shorter than any of the energy-containing scales in the inertial interval and it is determined by the most persistent scale in the flow, the scale of forcing. The above conclusion about the dominance in the diffusivity of one scale, which is close to the forcing scale, is at odds with results obtained in several studies, which find that the diffusivity is determined by the energy-containing eddy scales [20] , [21] , [22] , [23] . In 2D turbulence, in the presence of the inverse energy cascade, these scales are in the lower- k part of the Eulerian spectrum. The most likely reason for such discrepancy is the fact that in most models of turbulence (for example, Klocker et al . [23] ; Boffetta and Musacchio [24] ), forcing is defined as spatially periodic (localized in k ), but random in time (white noise). In these experiments, both in electromagnetically driven and in the Faraday waves driven turbulence, forcing scale vortices are substantially more coherent than turbulent eddies at any other scales. As discussed by Middleton [10] , the Lagrangian correlation function is related to the Eulerian spectrum via the modal correlation D ( k , t ) as . Here D ( k , t ) specifies the rate at which the motions of eddies of size k decorrelate with themselves. It is usually assumed that smaller scales decorrelate more rapidly (see for example, Middleton [10] ). This, however, is not true in these experiments where forcing is represented by a relatively narrow peak in the Lagrangian frequency spectrum shown in Fig. 4a . The spectrum F L ( f ) is computed as the ensemble averaged power spectrum of the Lagrangian velocity along the trajectory. A spectral peak around f =30 Hz is related to the forcing frequency, which in the case of the FWT is close to the Faraday frequency. The low frequency part of the spectrum, f <15 Hz corresponds to the Fourier transform of the temporal Lagrangian autocorrelation function ρ ( t ). 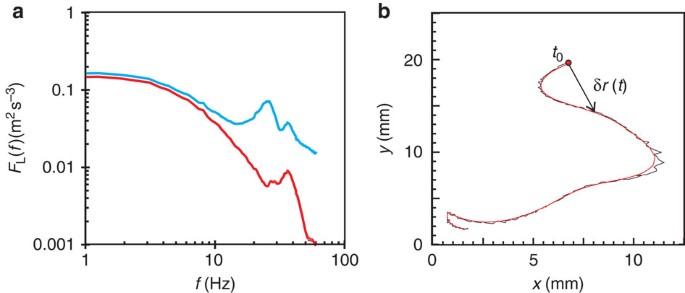Figure 4: Effects of trajectory smoothing. (a) Frequency spectrum of the Lagrangian velocity for the case of the FWT (vertical acceleration of 1.8g). The vertical vibration frequency isf0=60 Hz, corresponding to the Faraday frequency off=30 Hz. A peak atf≈30 Hz is due to forcing. Blue line corresponds to no smoothing of trajectories, red line corresponds to smoothing over one Faraday wave period. (b) Example of a particle trajectory: non-smoothed (black) and smoothed over one Faraday period trajectory (red). Figure 4: Effects of trajectory smoothing. ( a ) Frequency spectrum of the Lagrangian velocity for the case of the FWT (vertical acceleration of 1.8 g ). The vertical vibration frequency is f 0 =60 Hz, corresponding to the Faraday frequency of f =30 Hz. A peak at f ≈30 Hz is due to forcing. Blue line corresponds to no smoothing of trajectories, red line corresponds to smoothing over one Faraday wave period. ( b ) Example of a particle trajectory: non-smoothed (black) and smoothed over one Faraday period trajectory (red). Full size image Though Fig. 4a illustrates the coherency of forcing in these experiments, there can be other, perhaps more rigorous measures of the presence of persistent scales in a flow. For example, the persistence can be derived from the analysis of Lagrangian coherent structures using finite-time Lyapunov exponent field (see for example, Farazmand and Haller [25] and Ouellette [26] for additional comments on this). The lifetime of a persistent structure τ 0 can be determined by varying time interval of the Lyapunov exponent computation and comparing it with the turnover time of the turbulent eddy of size r in the Kolmogorov spectrum, τ r = ε −1/3 r 2/3 . A ratio τ 0 / τ r could be a measure of persistence of the scale r . A similar persistence parameter has been introduced in Sokolov [27] in the context of effects of coherent scales on the pair dispersion. It is possible that in some areas in the ocean forcing is correlated in time. This can be the case when small scale but coherent eddies are present (for example, Straneo et al . [28] ). In this case D ( k , t ) may be large for particular scales, which will greatly accentuate their role in the diffusivity. It is also useful to compute the Eulerian scale L E , defined as the integral of the Eulerian autocorrelation function of the velocity: Here the velocity is taken on a grid obtained from the particle image velocimetry (PIV) measurements rather than along the trajectories, and r 0 is taken in both the x and y directions. The Eulerian integral scale is determined as , or, if the autocorrelation function is approximately exponential, , it can be determined from the decay at short distances L . The Eulerian integral scale in the FWT is close to half the forcing scale, L E ≈(1/2) L f for different excitation frequencies (different L f ). A similar relation has also been mentioned in von Kameke et al . [15] This relation, together with the result of Fig. 3d , indicates that the Lagrangian correlation scale (or time) is not necessarily smaller than its Eulerian counterpart, L L ≤ L E , as it has been concluded from the theoretical analysis of Middleton [10] . In our case L L > L E , because the modal correlation D ( k , t ) in these experiments is different from those considered in Middleton [10] . Summarizing, the above results of laboratory studies of the tracer dispersion in 2D turbulence confirm that the diffusivity is determined as a product of the r.m.s. fluid particle velocity and the integral Lagrangian scale . This scale, which can be determined directly from the spatial Lagrangian velocity autocorrelation, equation (6), is related to the Lagrangian integral time, equation (4). The r.m.s. velocity depends on the kinetic energy accumulated in the turbulence inertial interval, and as such it is mostly determined by the energy-containing large scales. However, the scale L L that determines the diffusivity is not the energy-containing scale, but it is a smaller and less energetic, yet persistent scale determining the fluid particle's memory loss. In these experiments L L is related to the forcing scale. These results highlight the importance of coherent eddies in governing the diffusivity in turbulent flows and may appear useful in the analysis of the oceanic Lagrangian observations [29] . Turbulence generation To generate 2D turbulence, one needs to inject energy into the horizontal fluid motion at some intermediate range of scales, much smaller than the size of the container, and to ensure that this forcing is localized in the wave number domain to a relatively narrow band. Here turbulence is generated using two methods. In the first, EMT is produced in layers of electrolytes (here in Na 2 SO 4 water solution, specific gravity of SG=1.03) by running electric current J across the fluid cell [18] . A matrix of magnetic dipoles placed underneath the cell produces spatially varying magnetic field B . In these experiments 900 magnets were used (30 × 30 matrix, 10 mm between magnets). The Lorenz J × B force produces vortices, which drive turbulent flows. This corresponds to the forcing wave number of k f ≈ 630 m −1 . To reduce the bottom drag and to avoid the influence of the bottom boundary layer, a layer of electrolyte is placed on top of heavier (SG=1.8) non-conducting fluid (FC-3283 by 3 M) immiscible with water. Magnetic field at the interface between two layers is about B =0.3 T, while electric current density is changed in the range of J =(0.1–1.2) × 10 3 A m −2 . Green data points for EMT in Figs 2d and 3c correspond to the current densities of J =(0.1, 0.2, 0.4, 0.6, 0.8, 1.2) × 10 3 A m −2 from low to high < u 2 >, respectively. In the second method, the horizontal motion of fluid particles is forced by the parametrically excited Faraday waves on the surface of a vertically vibrated liquid (water) [15] , [16] . The floaters motion on the surface resembles the motion of fluid in 2D turbulence. This phenomenon is not restricted to thin layer of fluids, as was initially thought [15] , but it is also observed in deep (compared with Faraday wavelength) layers. The main advantage of generating turbulence using Faraday surface waves is the ability to change the forcing scale by simply changing the frequency of the vertical vibration. This method also allows a broader range of horizontal kinetic energies to be achieved [16] . In these experiments turbulence is generated in a circular container (180 mm diameter). In the wave number spectrum of kinetic energy, Fig. 1f , obtained at the vertical forcing frequency of 60 Hz, Kolmogorov k −5/3 spectrum is restricted at low k by the dissipation scale of about 200 m −1 . The dissipation prevents spectral condensation, or accumulation of spectral energy at the system scale. Measurements of single-particle dispersion have also been performed in a large square container (0.4 × 0.4 m 2 ) revealing no difference with the results reported here. However, at lower frequency excitation (30 Hz) in a smaller square container (0.1 × 0.1 m 2 ) spectral energy condenses into large coherent vortices [16] . Modifications to the fluid dispersion in this case will be reported elsewhere. Flow visualization and particle tracking The fluid motion is characterized using both PIV and particle tracking velocimetry techniques. In the EMT experiments, 50 μm diameter white polyamid particles (SG=1.03) are used. In the FWT experiments, black carbon glass particles are used to visualize fluid motion on the water surface. These particles have a diameter within a range of 150–300 μm (300 μm is the mesh size of the coarser sieve). The particles are plasma treated to reduce their intrinsic hydrophobicity. The use of surfactant and plasma treatment makes the particle wettability almost neutral, which prevents their clustering and insures homogeneous spreading on the fluid surface. Black particles are used in experiments where simultaneous visualization of Faraday waves (using diffusive light imaging) and floaters motion is needed, as described in Francois et al . [16] To test if the particle size (up to 300 μm) affects singe-particle dispersion, additional measurements are performed using 50 μm diameter white polyamid particles. No effect of the particle size is detected. This is consistent with observations [15] where 46 μm particles were used for PIV measurements and 300 μm particles were used for tracking Lagrangian trajectories. No differences were detected between the absolute dispersion derived from the 300 μm particle trajectories and the one computed using virtual tracers following the PIV velocity field. Previous studies of the finite particle size effects on transport in 2D flows demonstrated some inertial effects when the Stokes number St=(2/9)(ρ p /ρ f )( a / L ) 2 Re is relatively large, St ≥ 0.01 (ref. 30 ). Here ρ p and ρ f are the particle and fluid densities respectively, a is the particle radius and L is the characteristic flow length scale, and Re is the Reynolds number. In our experiments for the largest particles used ( a =0.15 mm) and the smallest forcing scale of L =3 mm, the Stokes number does not exceed St=5 × 10 −4 . In these conditions, finite particle size effects on single-particle dispersion can be neglected. The particle motion is captured using high-resolution fast camera (Andor Neo sCMOS). An example of a single-particle trajectory filmed in the FWT at the shaker excitation frequency of f 0 =60 Hz using camera's frame rate of 120 fps is shown in Fig. 4b . The trajectory is tracked using a nearest neighbour algorithm [31] . A maximum distance for the nearest neighbour search is set to be smaller than the minimal particle displacement between consecutive frames. A particle's position in Fig. 4b is recorded four times per period of the Faraday wave ( T F =2/ f 0 ). Orbital motion of a particle in the 3D surface ripple leads to the wiggles, or non-smoothness of the x – y trajectory (black). However, smoothing this trajectory over four points, or over T F restores smooth trajectory (red). 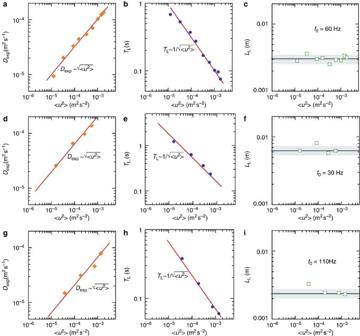Figure 5: Lagrangian statistics of single-particle dispersion in FWT. Diffusion coefficientDexp, Lagrangian integral timeTLand Lagrangian integral scaleLLversus velocity variance <u2> measured at different forcing frequencies: (a–c)f0=60 Hz, (d–f)f0=30 Hz, and (g–i)f0=110 Hz. Experimental data on particle dispersion Figure 5 shows the evolution of the diffusion coefficient D exp , Lagrangian integral time T L , and Lagrangian integral scale L L versus velocity variance in the Faraday waves driven turbulence at three different shaker frequencies. This data is used in the analysis of Figs 2 , 3 . Figure 5: Lagrangian statistics of single-particle dispersion in FWT. Diffusion coefficient D exp , Lagrangian integral time T L and Lagrangian integral scale L L versus velocity variance < u 2 > measured at different forcing frequencies: ( a – c ) f 0 =60 Hz, ( d – f ) f 0 =30 Hz, and ( g – i ) f 0 =110 Hz. Full size image How to cite this article: Xia, H. et al . Lagrangian scale of particle dispersion inturbulence. Nat. Commun. 4:2013 doi: 10.1038/ncomms3013 (2013).